Guided and magnetic self-assembly of tunable magnetoceptive gels Self-assembly of components into complex functional patterns at microscale is common in nature, and used increasingly in numerous disciplines such as optoelectronics, microfabrication, sensors, tissue engineering and computation. Here, we describe the use of stable radicals to guide the self-assembly of magnetically tunable gels, which we call ‘magnetoceptive’ materials at the scale of hundreds of microns to a millimeter, each can be programmed by shape and composition, into heterogeneous complex structures. Using paramagnetism of free radicals as a driving mechanism, complex heterogeneous structures are built in the magnetic field generated by permanent magnets. The overall magnetic signature of final structure is erased via an antioxidant vitamin E, subsequent to guided self-assembly. We demonstrate unique capabilities of radicals and antioxidants in fabrication of soft systems with heterogeneity in material properties, such as porosity, elastic modulus and mass density; then in bottom-up tissue engineering and finally, levitational and selective assembly of microcomponents. Self-assembly is a promising and non-invasive strategy for parallel fabrication of heterogeneous functional systems made of various microstructures [1] , [2] , [3] , [4] . Several self-assembly studies utilizing principles, such as fluidic force [5] , [6] , [7] , surface energy [8] , magnetic force [9] , [10] , gravity [11] , [12] , electrostatic force or capillary force [13] , [14] , [15] , have been presented for multiple applications [13] , [16] , [17] , [18] . These self-assembly methods are often massively parallel, and thus, less expensive and faster than deterministic methods such as robotic assembly. However, assembly precision and yield are not as high as serial pick-and-place assembly owing to the probabilistic nature of self-assembly. To increase the yield of the assembly, excessive number of components were used within the assembly regions [19] . Therefore, redundant mass fabrication of microstructures is required in most fluidic self-assembly methods, and there is an unmet need to develop efficient and inexpensive self-assembly methods merging the advantages of high-yield deterministic assembly and high-throughput self-assembly [20] . Microcomponent manipulation strategies using magnetics are versatile, contactless and inexpensive. In most of these strategies, magnetic micro/nano-beads are used [21] . Commercial magnetic beads are made of mainly iron oxide with minor amounts of other elements such as nickel and cobalt, encapsulated in a polymer shell. Because of the risk of heavy metal poisoning, use and release of such magnetic beads in clinical applications have to be proven. Therefore, alternative beads, potentially heavy metal-free, have to be developed for biological applications. The use of radicals with a purpose of leveraging their paramagnetism has not been well studied or broadly applied [22] , [23] , [24] , although it can provide a powerful tool to create magnetically responsive materials for manipulation of small building blocks for tissue engineering, and/or micro-manufacturing of soft systems. Herein, we present a broadly applicable strategy that allows fabrication of magnetically tunable microcomponents by stable radicals and vitamin E, and guide self-assembly of complex constructs in 3D with unique heterogeneous material properties such as porosity, elastic modulus and mass density. We use hydrogels as building blocks because of their advantageous biological properties, including moldability, high porosity and diffusion control [21] , [25] , [26] . Cells are reported to self-assemble and migrate in three-dimensional (3D) hydrogels in vitro [27] , [28] , [29] , [30] , [31] , [32] . Studies also show that migration behaviour of cells in 3D is different from that in two-dimensional (2D) [27] , [29] . In vivo , cells in functional units are embedded in a 3D microenvironment composed of extracellular matrix and neighbouring cells with a defined spatial distribution. Tissue functionality arises from these components and is influenced by their relative spatial locations [30] , [33] , [34] , [35] , [36] . When cells were cultured in 2D monolayers, they displayed significant difference in gene expression compared with cells in native tissues and in 3D culture conditions [37] . Hence, 2D systems do not effectively represent the complex 3D tissue environment [37] , [38] , [39] . The strategy here imparts hydrogels with features such as: (i) long magnetically active durations (up to 2 weeks), (ii) on/off magnetism by a simple and short antioxidant treatment when magnetization is no longer needed, (iii) no requirements for releasing of magnetic particles, that is, radicals can be quenched by vitamin E, compared with use of magnetic nanoparticles (MNPs) that need to be eliminated from the organism by physical release mechanisms through the kidney for clinical applications [40] , [41] . (iv) In addition, radicals are also used here to change magnetic signature of a microenvironment and selectively levitate and guide 3D self-assembly of microscale objects. Fabrication of magnetoceptive materials The principles that underlie the fabrication of magnetoceptive materials, and guided self-assembly of these components into complex structures are summarized in Fig. 1 . Photo-crosslinkable polymers methacrylated gelatin (GelMA) or polyethylene glycol dimethacrylate (PEGDMA) are used and crosslinked via ultraviolet (UV) light to fabricate microgels with patterned masks at scales of many hundreds of micrometre ( Fig. 1a ). To paramagnetize cell-encapsulating hydrogels, they are submerged into stable radical solution ( Fig. 1b ). Hydrogels are self-assembled with guidance of a permanent neodymium (NdFeB) magnet in a reservoir filled with an aqueous solution. The solution is composed of: (i) OptiPrep density gradient liquid to increase the density of solution enabling gels to float on the surface of the reservoir and (ii) surfactant Tween-80 to decrease the surface tension and drag forces on gels enabling faster motion of gels ( Fig. 1c ). When the distance between the magnet and hydrogel is decreased, the average velocity of hydrogel increases ( Supplementary Figs 1 and 2 ). To stabilize the overall shape of constructs, secondary crosslinking is performed following guided self-assembly. To switch off the magnetization of heterogeneous constructs and/or to minimize potential negative effects of free radicals on cell proliferation for tissue engineering applications, assembled constructs are submerged into vitamin E, an antioxidant solution, following the secondary crosslinking ( Fig. 1c , Supplementary Fig. 3 , Supplementary Note 1 ). Radicals are also utilized to change magnetic susceptibility of suspension liquid and to guide levitational self-assembly of beads and hydrogels ( Fig. 1d ). 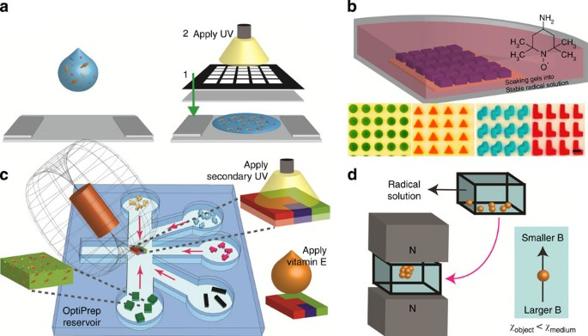Figure 1: Fabrication of magnetoceptive materials and guided self-assembly of microcomponents. (a) Microfabrication of cell encapsulating hydrogels via UV photocrosslinking. 50 μl of gel precursor solution was pipetted onto a glass slide, and then, exposed to UV light (500 mW; at a height of 50 mm above the gels) for 20 s. Several types of photomasks with different patterns were employed. (b) Submersion of cell encapsulating hydrogels into stable radical solution for paramagnetization. Inset: Micrographs of fabricated circular, triangular, zig-zag shaped and L-shaped hydrogel units. Scale bar is 1 mm. (c) Guided paramagnetic self-assembly of hydrogels using a permanent NdFeB magnet on a liquid reservoir composed of OptiPrep (20–30 (v/v) %) and Tween-80 (0.001 (v/v) %) in Dulbecco's Phosphate-Buffered Saline (DPBS). Following assembly, a minute amount of precursor solution is ejected onto the assembly. Secondary UV crosslinking was performed to stabilize the overall shape. Vitamin E treatment was applied to switch off the magnetism of assembled hydrogels, which in turn to increase the viability of cells that are encapsulated into hydrogels. (d) Levitational self-assembly of hydrogels in radical solution using two permanent NdFeB magnets in anti-Helmholtz configuration (same poles facing each other). Positive difference between magnetic susceptibilities of radical solution (χmedium) and gels (χobject) leads to levitational assembly of gels. Figure 1: Fabrication of magnetoceptive materials and guided self-assembly of microcomponents. ( a ) Microfabrication of cell encapsulating hydrogels via UV photocrosslinking. 50 μl of gel precursor solution was pipetted onto a glass slide, and then, exposed to UV light (500 mW; at a height of 50 mm above the gels) for 20 s. Several types of photomasks with different patterns were employed. ( b ) Submersion of cell encapsulating hydrogels into stable radical solution for paramagnetization. Inset: Micrographs of fabricated circular, triangular, zig-zag shaped and L-shaped hydrogel units. Scale bar is 1 mm. ( c ) Guided paramagnetic self-assembly of hydrogels using a permanent NdFeB magnet on a liquid reservoir composed of OptiPrep (20–30 (v/v) %) and Tween-80 (0.001 (v/v) %) in Dulbecco's Phosphate-Buffered Saline (DPBS). Following assembly, a minute amount of precursor solution is ejected onto the assembly. Secondary UV crosslinking was performed to stabilize the overall shape. Vitamin E treatment was applied to switch off the magnetism of assembled hydrogels, which in turn to increase the viability of cells that are encapsulated into hydrogels. ( d ) Levitational self-assembly of hydrogels in radical solution using two permanent NdFeB magnets in anti-Helmholtz configuration (same poles facing each other). Positive difference between magnetic susceptibilities of radical solution ( χ medium ) and gels ( χ object ) leads to levitational assembly of gels. Full size image Magnetic characterization of hydrogels To characterize the magnetization of hydrogels, electron paramagnetic resonance (EPR) measurements are performed ( Fig. 2 ). Cylindrical 20% (w/v) PEGDMA hydrogels are fabricated and soaked into phosphate-buffered saline (PBS; control), 10, 30 and 150 mg ml −1 stable radical solution. As the concentration of stable radical solution increases, EPR intensity or spin density, which is an indication of absorbed amount of radicals in hydrogels, increases ( Fig. 2a,b ). To show versatility of paramagnetization of hydrogels, we perform EPR measurements for 50% PEGDMA and 5% GelMA ( Fig. 2c–f ). Results show that 50% PEGDMA gels have the largest spin density indicating the highest absorbed amount of radicals among cases. Images of soaked hydrogels are given in Fig. 2b,d,f , respectively, which show a colour change depending on radical concentration. EPR spectra of all gels show an increase in spin density as the radical concentration increased ( Supplementary Note 2 ). Comparison of spin density after overnight soaking in stable radical solution is demonstrated in Fig. 2g . 50% PEGDMA shows the highest spin density. To switch off the paramagnetism, hydrogels are now ‘treated’ with an antioxidant vitamin E solution. We compare these hydrogel samples ( Fig. 2h ): (i) s1: PEGDMA gel soaked into radical solution, (ii) s2: PEGDMA gel soaked into radical solution, and then transferred into PBS (no vitamin E), and (iii) s3: PEGDMA gel soaked into radical solution, and then transferred into 0.5 mg ml −1 vitamin E, (+)-α-Tocopherol acetate, solution. Results show that spin density of vitamin E sample significantly decreased compared with the original sample ( Fig. 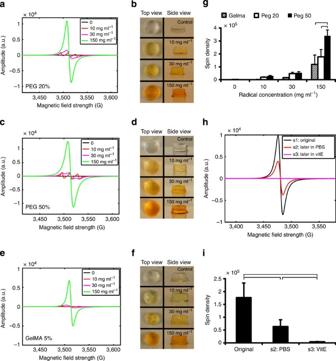Figure 2: Magnetic characterization of magnetically tunable hydrogels. Electron Paramagnetic resonance (EPR) spectra of 20% PEGDMA (a), 50% PEGDMA (c) and GelMA (e) soaked into PBS (control), 10, 30 and 150 mg ml−1(in PBS) stable radical solution for 10–15 h. Images of gels for a range of concentration. Top (left) and side (right) images of soaked 20% PEGDMA (b), 50% PEGDMA (d) and GelMA (f), which showed a colour change depending on radical concentration. Gels are cylindrical: 3 mm in diameter, 1.5 mm in height. EPR spectra has been performed with the sum of ten scans for each condition. Comparison of spin density in 20% PEGDMA, 50% PEGDMA and GelMA after overnight soaking in stable radical solution (g). Testing antioxidant vitamin E treatment (handi). EPR spectra (h) and spin densities (i) of samples s1, s2 and s3. Here s1 and s2 are controls, and s3 as the experiment sample. Sample s1: PEGDMA gel was soaked into radical solution. Sample s2: PEGDMA gel was soaked into radical solution, and then transferred into PBS (without vitamin E). Sample s3: PEGDMA gel was soaked into radical solution, and then transferred into 0.5 mg ml−1vitamin E, (+)-α-Tocopherol acetate. Spin densities were calculated computationally by integrating EPR spectra with trapezoidal rule. Horizontal lines connecting individual groups represent statistically significant difference (P<0.05). PEGDMA is abbreviated as PEG in the figure labels. Error bars represent s.d. from the mean (n=3–6). 2i ), indicating that the amount of free radicals are significantly decreased via antioxidant vitamin E. Figure 2: Magnetic characterization of magnetically tunable hydrogels. Electron Paramagnetic resonance (EPR) spectra of 20% PEGDMA ( a ), 50% PEGDMA ( c ) and GelMA ( e ) soaked into PBS (control), 10, 30 and 150 mg ml −1 (in PBS) stable radical solution for 10–15 h. Images of gels for a range of concentration. Top (left) and side (right) images of soaked 20% PEGDMA ( b ), 50% PEGDMA ( d ) and GelMA ( f ), which showed a colour change depending on radical concentration. Gels are cylindrical: 3 mm in diameter, 1.5 mm in height. EPR spectra has been performed with the sum of ten scans for each condition. Comparison of spin density in 20% PEGDMA, 50% PEGDMA and GelMA after overnight soaking in stable radical solution ( g ). Testing antioxidant vitamin E treatment ( h and i ). EPR spectra ( h ) and spin densities ( i ) of samples s1, s2 and s3. Here s1 and s2 are controls, and s3 as the experiment sample. Sample s1: PEGDMA gel was soaked into radical solution. Sample s2: PEGDMA gel was soaked into radical solution, and then transferred into PBS (without vitamin E). Sample s3: PEGDMA gel was soaked into radical solution, and then transferred into 0.5 mg ml −1 vitamin E, (+)-α-Tocopherol acetate. Spin densities were calculated computationally by integrating EPR spectra with trapezoidal rule. Horizontal lines connecting individual groups represent statistically significant difference ( P <0.05). PEGDMA is abbreviated as PEG in the figure labels. Error bars represent s.d. from the mean ( n =3–6). Full size image Magnetic responsiveness of hydrogels To show the versatility of the approach over different polymers, magnetic responsiveness of radicalized building units composed of PEGDMA and GelMA is evaluated ( Fig. 3 ). We keep hydrogels in radical solution for a range of concentrations 10, 30 and 150 mg ml −1 . Following fabrication of radicalized hydrogels, we keep hydrogels in a close proximity of NdFeB permanent magnet, and measure ‘magnetization time’, that is, the elapsed time until hydrogels are magnetized becoming responsive to a magnetic field by moving ( Fig. 3a ). Magnetically responsive hydrogels are counted within 15 s and 1 min, and their percentages are given in Fig. 3b, c , respectively. These results show that more than 90% of gels became magnetically responsive in 1 min. Then, to investigate the longevity of magnetic response of hydrogels, percentage of magnetically responsive gels is calculated for a range of incubation times: 0, 2, 5, 8 and 24 h ( Fig. 3d–f ). Results show that GelMA hydrogels remain magnetically responsive for a longer time ( Supplementary Fig. 4 ). Next, we increase the soaking time of hydrogels in stable radical solution to 1 day. Magnetization times and their deviations decrease as soaking concentration increases, indicating that gels become more responsive to magnetic field. 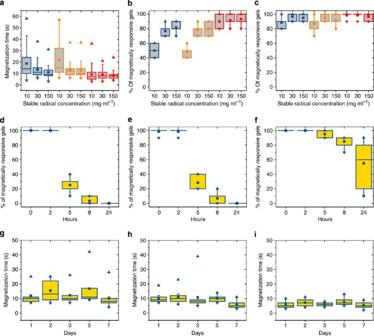Figure 3: Magnetic responsiveness of magnetically tunable hydrogels. (a) Magnetization time of radicalized hydrogels for 30 min. Magnetization time is the elapsed time until hydrogels were magnetized and became responsive to magnetic field. After applying (b) 15 s and (c) 1 min magnetic field, percentage of magnetically responsive hydrogels. Left to right in the plots (a–c): 20% PEGDMA (blue), 50% PEGDMA (orange) and 5% GelMA (red), respectively, for a range of stable radical concentration: 10, 30 and 150 mg ml−1. Gels are stained with 1% dye for 30 min, soaked in stable radical solution for another 30 min.n=10 measurements each. (d–f) Magnetic responsiveness of radicalized hydrogels: (d) 20% PEGDMA, (e) 50% PEGDMA and (f) 5% GelMA, for a range of elapsed time. Gels are stained with 1% dye for 30 min, soaked in stable radical solution for another 30 min.n=6 percentages, each percentage from ten measurements. (g–i) Magnetization time of radicalized 20% PEGDMA hydrogels for 1 day for a range of stable radical concentrations: (g) 10 mg ml−1, (h) 30 mg ml−1and (i) 150 mg ml−1.n=10 measurements each. Figure 3: Magnetic responsiveness of magnetically tunable hydrogels. ( a ) Magnetization time of radicalized hydrogels for 30 min. Magnetization time is the elapsed time until hydrogels were magnetized and became responsive to magnetic field. After applying ( b ) 15 s and ( c ) 1 min magnetic field, percentage of magnetically responsive hydrogels. Left to right in the plots ( a – c ): 20% PEGDMA (blue), 50% PEGDMA (orange) and 5% GelMA (red), respectively, for a range of stable radical concentration: 10, 30 and 150 mg ml −1 . Gels are stained with 1% dye for 30 min, soaked in stable radical solution for another 30 min. n =10 measurements each. ( d – f ) Magnetic responsiveness of radicalized hydrogels: ( d ) 20% PEGDMA, ( e ) 50% PEGDMA and ( f ) 5% GelMA, for a range of elapsed time. Gels are stained with 1% dye for 30 min, soaked in stable radical solution for another 30 min. n =6 percentages, each percentage from ten measurements. ( g – i ) Magnetization time of radicalized 20% PEGDMA hydrogels for 1 day for a range of stable radical concentrations: ( g ) 10 mg ml −1 , ( h ) 30 mg ml −1 and ( i ) 150 mg ml −1 . n =10 measurements each. Full size image Tunability of magnetoceptive materials Following characterization and quantification of paramagnetism, hydrogels are self-assembled with the guidance of magnetic field into heterogeneous patterns at the interface of liquid and air ( Fig. 4 , Supplementary Fig. 5 ). Rod and further complex assemblies composed of PEGDMA and GelMA hydrogels are depicted in Fig. 4a–e . To show patterning capability of such an on-demand strategy, hexagonal assemblies of PEGDMA hydrogels are performed at different configurations as shown in Fig. 4f–h . To show further complexity in assembly, gels are assembled into shapes given in Fig. 4i–k . Change in polymer concentration can change the contact angle between the suspending liquid and the hydrogel, and thus the meniscus forming between hydrogels in the assembly configuration, which in turn affects the gradients of liquid surface curvature and capillary forces ( Supplementary Fig. 6 ). Also, microcomponents can be programmed by composition, and heterogeneous assemblies of different polymers are formed ( Fig. 4l–n ). Then, we fabricate macroporous hydrogels by sucrose leaching [42] , and assemble them with nanoporous hydrogels into complex shapes ( Fig. 4o–q ). We also encapsulate glass bubbles (density=0.46 g cc −1 ) into gels to fabricate gels with lower mass density than normal glass-bubble-free gels ( Supplementary Fig. 7 ). Heterogeneous assemblies with varying mass densities (glass bubble encapsulating light PEGDMA gels and heavier PEGDMA gels together) are shown in Fig. 4r–t . To demonstrate the dynamic orientation control capability ( Supplementary Note 3 ) of our approach for manipulating and guiding assembly of a variety of microscale objects, we perform a tetris assembly. Image of the assembly, patterning setup and 3D sketch of tetris assembly are shown in Fig. 4u,v . Each well is used as a reservoir for different coloured hydrogels of various shapes: zig-zag, rod, square and T-polyomino. Snapshots of tetris assembly at different time points are given in Fig. 4w . 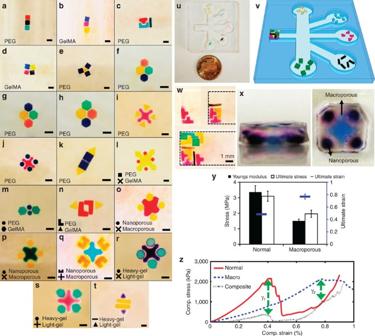Figure 4: Tunability of magnetoceptive materials. (a,b) Rod assemblies composed of PEGDMA and GelMA hydrogels. (c) Tetris-like assembly of PEGDMA. (d) Square assembly of GelMA. (e) Flower-like assembly of PEGDMA. (f–h) Hexagonal assembly of PEGDMA hydrogels. (i–k) More complex assemblies of PEGDMA hydrogels. (l–n) Heterogeneous assemblies consisting of both PEGDMA and GelMA. (o–q) Heterogeneous porous assemblies consisting of sucrose leached macroporous and nanoporous PEGDMA gels. (r–t) Assemblies with heterogeneity in mass density (glass bubble encapsulating light PEGDMA gels and heavier PEGDMA gels together). (u) Assembly and patterning setup with a penny. Each well is a reservoir for differently coloured hydrogels with different shapes. (v) 3D schematic of tetris patterning chamber. (w) Snapshots from tetris assembly at three time points (left to right). (x) 3D heterogeneous gel composed of three layers of macroporous (x-shape) and nanoporous (o-shape) 50% PEGDMA gels. From top view, gel cross-section is 5mm × 5mm. (y) Youngs Modulus, Ultimate Stress, and Ultimate Strain for normal and macroporous gels. Error bars represent s.e.m. (z) Compressive stress as a function of compressive strain for normal (solid), macroporous (dashed) and composite gels (dotted). PEGDMA is abbreviated as PEG in the figure labels. Scale bar is 1 mm. Figure 4: Tunability of magnetoceptive materials. ( a , b ) Rod assemblies composed of PEGDMA and GelMA hydrogels. ( c ) Tetris-like assembly of PEGDMA. ( d ) Square assembly of GelMA. ( e ) Flower-like assembly of PEGDMA. ( f – h ) Hexagonal assembly of PEGDMA hydrogels. ( i – k ) More complex assemblies of PEGDMA hydrogels. ( l – n ) Heterogeneous assemblies consisting of both PEGDMA and GelMA. ( o – q ) Heterogeneous porous assemblies consisting of sucrose leached macroporous and nanoporous PEGDMA gels. ( r – t ) Assemblies with heterogeneity in mass density (glass bubble encapsulating light PEGDMA gels and heavier PEGDMA gels together). ( u ) Assembly and patterning setup with a penny. Each well is a reservoir for differently coloured hydrogels with different shapes. ( v ) 3D schematic of tetris patterning chamber. ( w ) Snapshots from tetris assembly at three time points (left to right). ( x ) 3D heterogeneous gel composed of three layers of macroporous (x-shape) and nanoporous (o-shape) 50% PEGDMA gels. From top view, gel cross-section is 5mm × 5mm. ( y ) Youngs Modulus, Ultimate Stress, and Ultimate Strain for normal and macroporous gels. Error bars represent s.e.m. ( z ) Compressive stress as a function of compressive strain for normal (solid), macroporous (dashed) and composite gels (dotted). PEGDMA is abbreviated as PEG in the figure labels. Scale bar is 1 mm. Full size image 3D soft materials with multiple complex failure modes can have several applications in tissue engineering such as to investigate dynamic response of soft tissue surrogates during impact, or in soft robotics to create actuating or transmission components with different Young’s moduli. To show the 3D fabrication capability of our approach ( Supplementary Fig. 8 ), we first assemble gels into complex 2D shapes (step 1), then drain the solution out (step 2), then apply secondary crosslinking to stabilize the construct (step 3) and vitamin E treatment to switch off magnetization and recover any potential effect of radicals on cells (step 4). Then, we add embryo-tested mineral oil and OptiPrep solution (steps 5 and 6), which enables assembled gels to stay at the bottom of assembly chamber. Then, self-assembly of another set of gels is guided at the same location where the previous assembly is performed (step 7), and both liquids are drained out (step 8). This process is repeated one more time, and three-layered gel is fabricated ( Fig. 4x ). Then, we perform mechanical compression tests to determine Young’s Modulus of 20% PEGDMA gels (normal), sucrose-leached macroporous 20% PEGDMA gels and composite gels ( Fig. 4y ). Compressive stress versus compressive strain curves ( Fig. 4z ) show that the composite gels show two distinct failures, which particularly match with the ultimate strain of normal and macroporous gels. In addition, ultimate stress ( τ ) ratios at failure strains, that is, γ 1 = τ normal / τ composite and γ 2 = τ macroporous / τ composite are at the order of cross-section area ratios of normal and macroporous gels in the composite gels ( Fig. 4z ), which indicates that four columns (normal cylindrical gels) initially fail within the composite gel, and then remaining macroporous structure holds the integrity of composite gel until the secondary failure. Evaluation of cell viability and proliferation The organization and coding of cell-encapsulating hydrogels has broad applications in several fields including regenerative medicine, cell-based pharmaceutical research and tissue engineering [21] . The magnetic approach presented here offers a high level of control over complex tissue microenvironments. To show this capability, we evaluate the effects of stable radicals on cell viability and proliferation. Bright-field and fluorescence images of 3T3 cells encapsulated in GelMA hydrogels are shown at t =0, 3, 6 days for control group (no radical) and for radical group soaked into 30 mg ml −1 for 30 min ( Fig. 5a , top to bottom). Results show that 3T3 cells proliferated within all hydrogel groups including radical group ( Supplementary Fig. 9 ). Then, we perform MTT (3-(4,5-dimethylthiazol-2-yl)-2,5-diphenyl tetrazolium bromide) analysis to investigate proliferation of cells in the presence of radicals and vitamin E ( Fig. 5b–d ). Cell growth is plotted as a function of volume-to-volume ratios (v/v) of added radical suspension volume to cell suspension volume for days 0, 1, 3, 5 and 7, which shows proliferation of cells in the presence of stable radicals ( Fig. 5b , Supplementary Fig. 10 ). After paramagnetizing hydrogels via radicals (30 mg ml −1 for 30 min), exposing them to vitamin E solution for a range of vitamin E solution volume to cell suspension volume, results in increase of cell proliferation for >50% (v/v) vitamin E solution ( Fig. 5c ). To investigate the effects of stable radicals on cell viability and proliferation, we first evaluate cell viability for a range of radical concentrations: 10, 30 and 150 mg ml −1 , keeping vitamin E solution constant at 100% (v/v). Results show that for large concentration of radical, for example, 150 mg ml −1 (and for 30 min incubation), vitamin E does not significantly help to recover cells. Faster actuation of radical-impregnated hydrogels requires higher concentrations of radicals, which in turn are more difficult to be quenched by vitamin E. Cell growth and functionality are reduced significantly when high concentrations of radicals (150 mg ml −1 ) are utilized for magnetization of hydrogels. We show viabilities of 3T3 cells after we assembled gels into square, rod-shaped and L-shaped constructs ( Fig. 5e ). We isolate and encapsulate primary cardiomyoctes into GelMA gels ( Fig. 5f,g , Supplementary Fig. 11 ). Results are shown for: (f) control (no radical) and (g) × 40 magnification of gels exposed to radicals and vitamin E. Cells are stained with mouse anti-α-actinin (sarcomeric) and anti-GATA-4. Actin cytoskeleton is visualized with phalloidin and 4′,6-diamidino-2-phenylindole (DAPI) is used as nuclear counter staining. Results show that cardiomyoctes preserve their phenotypic properties and functionalities after radical exposure and vitamin E recovery at day 10. 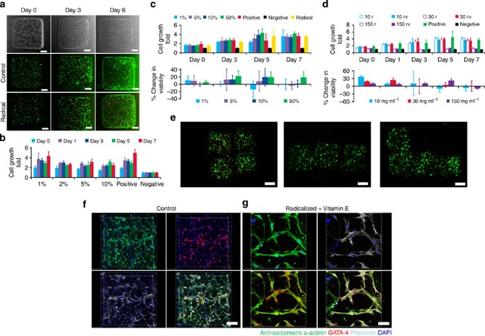Figure 5: Evaluation of cell viability and proliferation in the presence of stable radicals. (a) Bright-field (control) and fluorescence images of 3T3 cells encapsulated in GelMA hydrogels were shown att=0, 3, 6 days (top to bottom) for control group (no radicals) and for radical group soaked into 30 mg ml−1for 30 min. Green represented live cells and red represented dead cells. (b) MTT (3-[4,5-dimethylthiazol-2-yl]-2,5 diphenyl tetrazolium bromide) assay results as a function of volume-to-volume ratios (v/v) of added radical suspension volume to cell suspension volume for days 0, 1, 3, 5 and 7. The histograms showed proliferation of cells in the presence of stable radicals. Positive control represents cells without radicals. Negative control is only the MTT reagents. All results were normalized with respect to negative control. Error bars represent s.e.m. (c) After paramagnetizing hydrogels via radicals (30 mg ml−1for 30 min), exposing them to vitamin E solution resulted in increase of cell proliferation for >50% (v/v) vitamin E solution. Results were given for a range of vitamin E solution volume to cell suspension volume. Error bars represent s.e.m. (d) After paramagnetizing hydrogels via radicals for a range of radical concentration (10, 30, 150 mg ml−1), exposing them to vitamin E solution (100% (v/v)). Labels with ‘r’ in the figure caption, such as ‘10 r’, corresponds to hydrogels radicalized with 10 mg ml−1, and labels with ‘rv’ corresponds to gels exposed to vitamin E following radicalization. Results showed that for large concentration of radical, for example, 150 mg ml−1(and for 30 min incubation), vitamin E does not significantly help to recover cells. Error bars represent s.e.m. (e) Fluorescent images of square, rod-shaped and L-shaped assemblies of 3T3 encapsulating GelMA hydrogels. Scale bars are 200 μm. (f,g) Cardiomyocyte encapsulating GelMA hydrogels: (f) control (no radicals), (g) × 40 magnification of radical and vitamin E exposed gels. Scale bars are 200 μm (f) and 100 μm (g). Cells were stained with mouse anti-α-actinin (sarcomeric) and anti-GATA-4. Actin cytoskeleton was visualized with phalloidin and DAPI was used as nuclear counter staining. All images were shown on day 10. Figure 5: Evaluation of cell viability and proliferation in the presence of stable radicals. ( a ) Bright-field (control) and fluorescence images of 3T3 cells encapsulated in GelMA hydrogels were shown at t =0, 3, 6 days (top to bottom) for control group (no radicals) and for radical group soaked into 30 mg ml −1 for 30 min. Green represented live cells and red represented dead cells. ( b ) MTT (3-[4,5-dimethylthiazol-2-yl]-2,5 diphenyl tetrazolium bromide) assay results as a function of volume-to-volume ratios (v/v) of added radical suspension volume to cell suspension volume for days 0, 1, 3, 5 and 7. The histograms showed proliferation of cells in the presence of stable radicals. Positive control represents cells without radicals. Negative control is only the MTT reagents. All results were normalized with respect to negative control. Error bars represent s.e.m. ( c ) After paramagnetizing hydrogels via radicals (30 mg ml −1 for 30 min), exposing them to vitamin E solution resulted in increase of cell proliferation for >50% (v/v) vitamin E solution. Results were given for a range of vitamin E solution volume to cell suspension volume. Error bars represent s.e.m. ( d ) After paramagnetizing hydrogels via radicals for a range of radical concentration (10, 30, 150 mg ml −1 ), exposing them to vitamin E solution (100% (v/v)). Labels with ‘r’ in the figure caption, such as ‘10 r’, corresponds to hydrogels radicalized with 10 mg ml −1 , and labels with ‘rv’ corresponds to gels exposed to vitamin E following radicalization. Results showed that for large concentration of radical, for example, 150 mg ml −1 (and for 30 min incubation), vitamin E does not significantly help to recover cells. Error bars represent s.e.m. ( e ) Fluorescent images of square, rod-shaped and L-shaped assemblies of 3T3 encapsulating GelMA hydrogels. Scale bars are 200 μm. ( f , g ) Cardiomyocyte encapsulating GelMA hydrogels: ( f ) control (no radicals), ( g ) × 40 magnification of radical and vitamin E exposed gels. Scale bars are 200 μm ( f ) and 100 μm ( g ). Cells were stained with mouse anti-α-actinin (sarcomeric) and anti-GATA-4. Actin cytoskeleton was visualized with phalloidin and DAPI was used as nuclear counter staining. All images were shown on day 10. Full size image Levitational and guided self-assembly using radicals Aqueous solutions of gadolinium (Gd 3+ ) and manganese (Mn +2 ) ion salts have been widely used for levitation of beads and particles [43] . Here, we explore the use of radicals in levitational guided self-assembly of soft and rigid objects. A magnetic setup composed of two permanent NdFeB magnets in anti-Helmotz configuration (like poles facing each other) is fabricated ( Supplementary Fig. 12 ) to levitate microcomponents. The simulation of magnetic field norm (contour) and flux density (arrows) created by the magnetic setup ( Fig. 6a ) shows that magnetic field is minimum at the centre of symmetry axes ( Supplementary Fig. 13 , Supplementary Note 4 ). Then, we suspend 1 cm × 1 cm × 1.5 mm 20% PEGDMA hydrogel into a radical solution ( Fig. 6b ) and place the reservoir into the magnetic setup ( Fig. 6c ), which results in levitation of hydrogel because of the paramagnetism of radical solution ( Supplementary Movie 1 ). To illustrate the competing effects in the presence of both radicals and conventionally used ion salts, we prepare two samples: non-radicalized hydrogel (gel at left, Fig. 6d ) and radicalized hydrogel (gel at right, Fig. 6d ) and place them into Gadolinium (Gd) solution. Non-radicalized hydrogel that does not have a significant magnetic signature levitates because of the paramagnetism of Gd solution. On the other hand, the radicalized hydrogel does not levitate due to cancelling effects among paramagnetisms of radicals and Gd ion salts ( Fig. 6e , Supplementary Movie 2 ). Then we use smaller and multiple gels of each type (radicalized and non-radicalized) to demonstrate selective assembly of gels. Radicalized hydrogels (blue) do not levitate because of cancelling effects between paramagnetism of radicals and Gd ion salts, whereas non-radicalized hydrogels (yellow) are levitated and assembled because of paramagnetism of Gd solution ( Fig. 6f,g , Supplementary Movie 3 ). Finally, 500 μm polystyrene beads are used to quantify temporal changes of the assembly areas in Gd and radical solutions ( Fig. 6h , Supplementary Movies 4 and 5 ). Snapshots are given before ( Fig. 6i ) and after ( Fig. 6j ) assembly in radical solution. Increase in the distance between two magnets lead to an increase in levitation height of beads in radical solution ( Supplementary Figs 14 and 15 ). 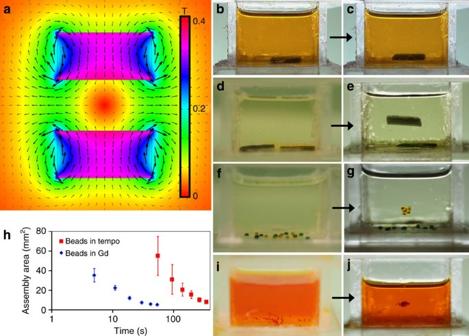Figure 6: Levitational and guided self-assembly of micro-components using radicals. (a) Simulation of magnetic field norm (contour) and flux density (arrows) created by two magnets in anti-Helmholtz configuration. (b,c) 1 × 1 cm220% PEGDMA hydrogels in a radical solution reservoir; before (b) and after (c) being placed into a magnetic setup composed of permanent NdFeB magnets in anti-Helmholtz configuration (same poles facing each other). Hydrogels are levitated due to the paramagnetism of radical solution. (d,e) Non-radicalized (left) and radicalized (right) 1 × 1 cm2hydrogels in Gadolinium (Gd) solution; before (d) and after (e) being placed into magnetic setup. Radicalized hydrogel did not levitate because of cancelling effects between paramagnetism of radicals and Gd ion salts, whereas non-radicalized hydrogel levitated because of paramagnetism of Gd solution. (f,g) Non-radicalized (yellow) and radicalized (blue) 1 × 1 mm2hydrogels in Gd solution; before (f) and after (g) being placed into the magnetic setup. Radicalized hydrogels (blue) did not levitate because of cancelling effects between paramagnetism of radicals and Gd ion salts, whereas non-radicalized hydrogels (yellow) were levitated and assembled because of the paramagnetism of Gd solution. (h–j) Levitational guided self-assembly of 500 μm polystyrene beads. Quantification of assembly areas as a function of time for beads in Gd and radical solution (h). Error bars represent s.d. from the mean. Snapshots are given before (i) and after (j) assembly in radical solution. Figure 6: Levitational and guided self-assembly of micro-components using radicals. ( a ) Simulation of magnetic field norm (contour) and flux density (arrows) created by two magnets in anti-Helmholtz configuration. ( b , c ) 1 × 1 cm 2 20% PEGDMA hydrogels in a radical solution reservoir; before ( b ) and after ( c ) being placed into a magnetic setup composed of permanent NdFeB magnets in anti-Helmholtz configuration (same poles facing each other). Hydrogels are levitated due to the paramagnetism of radical solution. ( d , e ) Non-radicalized (left) and radicalized (right) 1 × 1 cm 2 hydrogels in Gadolinium (Gd) solution; before ( d ) and after ( e ) being placed into magnetic setup. Radicalized hydrogel did not levitate because of cancelling effects between paramagnetism of radicals and Gd ion salts, whereas non-radicalized hydrogel levitated because of paramagnetism of Gd solution. ( f , g ) Non-radicalized (yellow) and radicalized (blue) 1 × 1 mm 2 hydrogels in Gd solution; before ( f ) and after ( g ) being placed into the magnetic setup. Radicalized hydrogels (blue) did not levitate because of cancelling effects between paramagnetism of radicals and Gd ion salts, whereas non-radicalized hydrogels (yellow) were levitated and assembled because of the paramagnetism of Gd solution. ( h – j ) Levitational guided self-assembly of 500 μm polystyrene beads. Quantification of assembly areas as a function of time for beads in Gd and radical solution ( h ). Error bars represent s.d. from the mean. Snapshots are given before ( i ) and after ( j ) assembly in radical solution. Full size image By guiding the self-assembly of the building units at the air–fluid interface paramagnetically or within the radical medium diamagnetically, it is possible to pattern multicomponent structures, which can differentiate among each other by shape, colour and material properties such as mass density, elastic modulus and porosity ( Supplementary Note 5 ). Magnetization of microcomponents via free radicals is a versatile and robust strategy, as several sub-processes such as staining, cell encapsulation or engineering macroporosity can be performed before radical exposure of gels for magnetization. On the other hand, MNP encapsulating hydrogels has to be fabricated by mixing MNPs with prepolymer solution [40] and cell suspension before cross-linking step, thus during further steps, such as long leaching times (several hours [42] ) of engineering macroporosity, cells are exposed to toxic MNPs. There is also limited control over release of MNPs, and no guarantee on cleansing of MNPs from scalable large tissue constructs generated by MNP-assembly method [40] , [44] . A multiplicity of antioxidants (such as a combination of vitamin E, vitamin C, glutathione, gamma-tocopherol, melatonin, lycopene) can be used to increase effectiveness of antioxidant treatment because different antioxidants are particularly effective for neutralizing specific reactive oxygen species (ROS) or reactive nitrogen species (RNS) [45] . Stable radical-impregnated hydrogels allow more stable and robust actuation compared with hydrogels magnetized via free radicals because of UV fabrication [10] . Radical formation during the UV crosslinking step were not controllable or stable to enable significant applications [10] . Their formation, quenching, presence or concentration cannot be controlled becauase of their random and non-stable nature [10] . In our earlier work [10] , a portion of hydrogels were magnetically active after UV fabrication owing to faster decay of free radicals and random formation, which decreased throughput of the approach. In addition, longer UV crosslinking times (for example, 100 s) were required for more random formation of radicals, which led to easier and faster manipulation of gels. This increase in crosslinking time in turn was more harmful to cells. Here we showed that use of stable radicals with an anti-oxidant treatment can be applied to material fabrication with numerous applications. Initially, we envision non-invasive applications in pharmaceutical or drug testing. In addition, radicals can be encapsulated into shell or capsules, and the interaction between cells and radicals can be further minimized by such barriers, which may potentially require an optimization step to minimize magnetic interference or dilution that might be caused by barrier itself. The presented approach here leveraging the magnetism of radicals, can also open a new field for engineering radicals with superior magnetism. In summary, we have demonstrated a new approach to fabricate magnetically tunable materials and guide the self-assembly of such soft living structures into complex constructs with unique spatially heterogeneous material properties including mass density, porosity and elastic modulus. We also showed selective levitational assembly of microcomponents utilizing stable radicals. A variety of 2D and 3D self-assembled structures can be generated by inexpensive permanent magnets without external power, and in an environment free of solid–solid contact. Our work gives new insights into the use of free radicals and antioxidants for magnetic actuation, guided self-assembly and erasing magnetic signature of such living microscale building blocks for scalable and parallel material synthesis. In addition to tissue engineering, this approach can be used to build biologically active, soft 3D hydrogel constructs to be employed in soft robotics, or heterogeneous microphysiological systems for pharmaceutical research and diagnostics. Fabrication of microgels PEGDMA microgel prepolymer solution was prepared by dissolving poly(ethylene glycol) 1000 dimethacrylate (PEGDMA; Polysciences, Inc.; 20%, 50% (w/v)) in PBS (Gibco; 1 ml). Photoinitiator (PI) 2-hydroxy-1-(4-(hydroxyethoxy)phenyl)-2-methyl-1-propanone (1%, w/v, Irgacure 2959; CIBA Chemicals) was then added to the prepolymer solution. 40 μl PEGDMA prepolymer solution was pipetted between spacers (coverslip 25 × 25 mm 2 , thickness: 150 μm) on the backside of 95 × 15 mm 2 Pyrex reusable Petri dish (Fisher Scientific). Another coverslip was placed onto the droplet. A photomask (1 × 1 mm 2 ; square) was set on the coverslip between the UV light and prepolymer droplet. Microgels were fabricated by applying UV light (6.9 W cm −2 ; at a height of 50 mm above the microgels) for 30 s. Then, photomask and coverslip were removed, and square PEGDMA microgels were formed on the coverslip. By using a razor (American Safety Razor, American Line), the microgels were transferred into PBS filled assembly chambers. GelMA microgel prepolymer solution was prepared by dissolving gelatin methacrylate lyophilized powder (5% (w/v)) in PBS (Gibco; 1 ml). Then, PI 2-hydroxy-1-(4-(hydroxyethoxy)phenyl)-2-methyl-1-propanone (0.5%, w/v, Irgacure 2959; CIBA Chemicals) was added to the prepolymer solution. A 40 μl droplet of GelMA prepolymer solution was pipetted onto the backside of 80 × 15 mm 2 Pyrex reusable Petri dish (Fisher Scientific) between spacers (cover slip 25 × 25 mm 2 , thickness: 150 μm). A photomask (1 × 1 mm 2 ; square) was set on the coverslip between the UV light and prepolymer droplet, after another coverslip was placed onto the droplet. Microgels were fabricated by applying UV light (2.9 W cm −2 ; at a height of 50 mm above the microgels) for 30 s. Then, photomask and coverslip were removed, and square GelMA microgels were formed on the coverslip. By using a razor, the microgels were transferred into PBS filled assembly chambers. Radicalized PEGDMA hydrogel fabrication for EPR measurements A coverslip was placed under poly(methyl methacrylate) (PMMA) mold (PMMA; 1.5 mm height; 3 × 3 cm 2 , square) with a cavern (3 mm diameter; circular) in the centre. Then, cylindrical PEGDMA gel was fabricated by filling PEGDMA prepolymer solution (PEGDMA 1000 with 1% PI; and two cases: 20 and 50% (w/v) dissolved into PBS) into the mold. Then, another coverslip was placed onto PMMA mold. UV light (6.9 W cm −2 ; at a height of 50 mm above the mold) was applied for 30 s. Stable radical 4-Amino-2,2,6,6-Tetramethylpiperidine-1-oxyl (4-Amino-Tempo; Sigma; 10 mg; 30 mg ml −1 ; 150 mg) solution was prepared by dissolving stable radical powder into PBS (Gibco; 1 ml). Then, after coverslips were removed, solid cylindrical PEGDMA gel was obtained. Stable radical solution (10, 30, 150 mg dissolved into 1 ml PBS). Then, four cylinder PEGDMA hydrogels were separated into control and experimental groups by following experiments: (i) Control: place a PEGDMA hydrogel into a 35 × 10 mm 2 Pyrex reusable Petri dish (Fisher Scientific) filled with 1 ml PBS for 10 h, (ii) Experiment A: place a PEGDMA hydrogel into a Petri dish filled with 10 mg ml −1 stable radical solution for 10 h, (iii) Experiment B: place a PEGDMA hydrogel into a Petri dish filled with 30 mg ml −1 stable radical solution for 10 h, (iv) Experiment C: place a PEGDMA hydrogel into a Petri dish filled with 150 mg ml −1 stable radical solution for 10 h. Four PEGDMA hydrogels were then placed into the tubes for EPR measurements. Please note that here and in the next sections, 10 h refer to overnight incubation. Vitamin E-treated PEGDMA hydrogel fabrication for EPR A coverslip was placed under PMMA mold (1.5 mm height; 3 × 3 cm 2 , square) with a cavern (3 mm diameter; circular) in the centre. Cylindrical PEGDMA gel was fabricated by filling PEGDMA prepolymer solution (PEGDMA 1000 with 1% PI; 50% (w/v) dissolved into PBS) into the mold. Then, another coverslip was placed onto PMMA mold. UV light (6.9 W cm −2 ; at a height of 50 mm above the mold) was applied for 30 s to achieve crosslinking within photo-crosslinkable PEGDMA prepolymer solution. After coverslips were removed, solid cylindrical PEGDMA gel was obtained. Stable radical (4-Amino-Tempo; Sigma) solution (10, 30, 150 mg dissolved into 1 ml PBS). PEGDMA hydrogels were separated into control and experimental groups: (i) Experiment: place a PEGDMA hydrogel into a 35 × 10 mm 2 Pyrex reusable Petri dish (Fisher Scientific) filled with 150 mg ml −1 stable radical for 10 h. Then, PEGDMA hydrogel was taken out, washed with 1 ml PBS for three times and soaked into 0.05% (w/v) water soluble vitamin E ((+)-α-Tocopherol acetate; Sigma) dissolved in PBS (Sigma) for another 10 h. (ii) Control A: place a PEGDMA hydrogel into Petri dish filled with 150 mg ml −1 stable radical solution for 10 h. (iii) Control B: place a PEGDMA hydrogel into a 35 × 10 mm 2 Petri dish filled with PBS for 10 h. Media preparation for paramagnetic floating of hydrogels For PEGDMA gel assemblies, media for paramagnetic floating of hydrogels was prepared by using 20% (v/v) OptiPrep (Optiprep Density Gradient Medium; Sigma; blending with PBS). Then, 0.001% (v/v) Tween-80 (Tween 80 viscous liquid; Sigma) was added into the solution. For GelMA hydrogel assemblies, media for paramagnetic floating of hydrogels was prepared by using 30% (v/v) OptiPrep (Optiprep Density Gradient Medium; SIGMA; blending with PBS). Then, 0.001% (v/v) Tween-80 (Tween 80 viscous liquid; SIGMA) was added into the solution. Cell viability and proliferation assays NIH 3T3 cells were cultured in Dulbecco’s modified Eagle’s medium (Invitrogen) supplemented with 10% fetal bovine serum (Invitrogen) and 1% penicillin–streptomycin (Gibco) mixture in a humidified and 5% CO 2 containing atmosphere at 37 °C. For MTT (Mw=414) viability assay (Invitrogen), cells were seeded in a 96-well plate with the density of 10 5 cells per ml (a total volume of 100 μl cell suspension per well). Stable radical 4-Amino-TEMPO solutions were prepared with the concentrations of 10, 30, 90 and 150 mg ml −1 . When the cells were attached after 4 h, stable radical solutions were added to the wells in different amounts (1, 2, 5, 10 and 20% (v/v)). The cells were incubated with stable radical solution for 30 min at 37 °C. After 30 min, stable radical containing cell culture medium was aspirated from the wells for all samples. Positive control samples were the samples that were not incubated with stable radical. Then fresh culture medium and MTT reagent (10% (v/v)) were added to all wells and incubated for 2 h. At the end of 2 h, resulting formazan was dissolved in 100 μl MTT solubilizing reagent SDS (Mw=288). Absorbance of induced formazan dye was measured by BMG FLUOstar Galaxy—Multi-functional Microplate Reader on the next day. All determinations were carried out in six repeats for each sample and three independent experiments were carried out. MTT proliferation assays were performed 0, 1, 3, 5 and 7 days after the addition of the 4-Amino-TEMPO solution on the cells. Vitamin E treatment for MTT assay To recover the potential negative effects of stable radicals on cells, vitamin E treatment was performed. Vitamin E solution in sterile PBS was prepared with the maximum solubility of 0.5 mg ml −1 . Following stable radical incubation, vitamin E solution was added to the wells in different volume ratios as such 1, 5, 10 and 50% (v/v) and cells were incubated for 30 min. After 30 min, vitamin E containing culture medium was aspirated and MTT assay was performed. Another vitamin E treatment was performed by adding 100% (v/v) vitamin E solution to the wells for 30 min after stable radical incubation. The effect of vitamin E treatment on the viability of 3T3 cells was analysed by MTT assay for days 0, 1, 3, 5 and 7. 3T3 cell encapsulation and live/dead assay The cover slides used for microgel fabrication were coated with 3-(trimethoxysilyl)propyl methacrylate (TMSPMA, Sigma) as previously described [7] . The secondary coating was applied on the cover slides with 20% (w/v) PEGDMA (2% (w/v) PI). GelMA 5% (w/v) prepolymer solution was prepared by first dissolving the 0.5% (w/v) PI in PBS. When the PI was dissolved completely, lyophilized gelatin methacrylate 5% (w/v) was added and dissolved at 80 ° C. 3T3 cells were resuspended in prepolymer solution at room temperature (RT) with a cell density of 5 × 10 6 cells per ml right before the encapsulation step. 40 μl of cell suspension in prepolymer solution was placed on a TMSPMA and PEGDMA-coated glass slide and photo-crosslinking was performed under UV light 2.6 mW cm −2 for 25 s (Omnicure S2000). 1 × 1 mm 2 cell encapsulating hydrogels were obtained. Cell-laden hydrogels were washed with PBS to remove any remaining prepolymer solution and submerged in culture media and cultured in an incubator (5% CO 2 , 37 °C) for 4 h. Following the 4 h incubation time, cells were incubated with 30 mg ml −1 5% (v/v) stable radical solution for 30 min and washed. Live/Dead viability assay (Molecular Probes, Invitrogen) was performed for Day 0 samples. Culture media was removed and 150 μl of Live/Dead assay reagent was added to the surface of the microgels and incubated for 20 min at 37 °C. Live/Dead dyes were prepared by adding 20 μl of the supplied 2 mM Ethidium homodimer-1 (EthD-1, Molecular Probes) stock solution to 10 ml sterile PBS and vortexed. Then 5 μl of the supplied 4 mM calcein AM stock solution was combined with EthD-1 solution and vortexed again. The living encapsulated cells were labelled green with Calcein AM and the dead cells were labelled red with EthD-1 linker. The florescent images were taken using an inverted fluorescent microscope (Carl-Zeiss AXIO). The viability of the encapsulated cells was quantified with Image J ITCN (Image based tool for counting nuclei) cell counting plug-in. Immunocytochemistry staining 3T3 cells encapsulating gels were fixed with 4% paraformaldehyde for 20 min at RT and washed. Gels were permeabilized with 0.3% Triton-X 100 (Sigma), in 1% bovine serum albumin (BSA) (Sigma), for min 2 h at RT. Gels were stained with rabbit anti Ki67 (Ab16667, Abcam) overnight at 4 °C. Following the washing step gels were incubated with secondary antibody goat anti-rabbit Alexa Fluor 564 (A11011, Invitrogen) for 2 h at RT. DAPI was used as nuclear counter staining. After washing, hydrogels were visualized under fluorescent microscope (Carl-Zeiss AXIO). Rat heart dissection and cadiomyocyte isolation Complete growth medium consisted of Dulbecco’s modified Eagle’s medium (Gibco), 10% horse serum (Gibco), 2.5% fetal bovine serum (Gibco), 100 U ml −1 penicillin and 100 mg ml −1 streptomycin (Gibco). 0.1% (w/v) collagenase type II enzyme (270 U mg −1 , Worthington Biochemical) was used to dissociate pieces of heart tissue into single cells. One- to two-day old Sprague–Dawley rats were used for isolation of neonatal cardiomyocytes. Rats were dissected according to the Institutional Animal Care and Use Committee at the Harvard Medical School, under an approved protocol #04821. Hearts were rinsed in ice-cold Hank's Balanced Salt Solution (HBSS) buffer (Ca 2+ - and Mg 2+ -free, Corning Cellgro) to remove blood cell components. They were minced with scissors into 1–2 mm 3 pieces into ice-cold HBSS. The minced ventricles were placed in 0.1% (w/v) purified trypsin (Gibco) in ice-cold HBSS for 15–18 h at 4 °C at low-speed shaker. Complete growth medium was added to inhibit trypsin digestion and waited at 37 °C for 5 min. Pieces of heart tissue were incubated with collagenase solution for digestion at 37 °C. Incubations were done with collagenase five times (10 min each) and first cell suspension was aspirated to remove dead and damaged cells, debris and blood cells. The collected cell suspensions were passed through a 70-μm cell strainer. Cells were centrifuged at 1,000 r.p.m. for 5 min to remove collagenase. After resuspension in warm complete growth medium, cells were pre-plated for 60 min to enrich cardiac myocytes. After counting cells, the cell suspension was adjusted to a concentration of 1 × 10 6 cells in 1 ml GELMA prepolymer solution. Cardiac cell encapsulation TMSPMA and 20% (w/v) PEGDMA-coated glass slides were prepared before the cardiomyocyte encapsulation and microgel fabrication. GelMA 3% (w/v) prepolymer solution was prepared by first dissolving the PI 0.1% (w/v) in PBS. When the PI is dissolved completely, lyophilized gelatin methacrylate 3% (w/v) was added and dissolved at 80 °C. Primary cardiomyocytes were counted and then resuspended in GelMA 3% (w/v) prepolymer solution with a cell density of 10 × 10 6 cells per ml right before the encapsulation step. 40 μl of cell suspension in prepolymer solution was placed on a TMSPMA and PEGDMA-coated glass slide and photo-crosslinking was performed under UV light 2.9 mW cm −2 for 25 s (Omnicure S2000). 1 × 1 mm 2 cell encapsulating hydrogels were obtained by UV photo mask. Cell-laden hydrogels were washed with PBS to remove any remaining prepolymer solution and submerged in culture media then cultured in an incubator (5% CO 2 , 37 °C) for 4 h. Following the 4 h incubation time, cells were incubated with 10 and 30 mg ml −1 5% (v/v) stable radical 4-Amino-TEMPO solution for 30 min and then washed. Vitamin E treatment Following stable radical incubation, 0.5 mg ml −1 vitamin E solution in culture medium was added to the wells in a concentration of 100% (v/v) and then incubated for 30 min. After 30 min, vitamin E containing culture medium was aspirated and encapsulated cells were further cultured for 10 days. Immunocytochemistry staining Cardiomyocyte encapsulating hydrogels were fixed with 4% paraformaldehyde for 20 min at RT and washed with PBS. Gels were blocked in 1% BSA (Sigma) and permeabilized with 0.3% Triton-X 100 (Sigma) for min 2 h at RT. Cells were stained with mouse anti-α-actinin (sarcomeric; A7811, Sigma) and rabbit anti-GATA-4 (ab5245, Abcam) for overnight at 4 °C. Samples were washed and stained for secondary goat anti-mouse Alexa Fluor 488 and goat anti-rabbit Alexa Fluor 568 antibodies (Life Technologies) for 2 h at RT. Actin cytoskeleton was visualized with Alexa Fluor 647 phalloidin (Life Technologies) and DAPI was used as nuclear counter staining. After washing, hydrogels were visualized with Leica SP8 X inverted confocal microscope (Leica). Gel fabrication for levitation experiments Gel fabrication for Supplementary Movie 1 . Pyrolytic graphite-embedded PEGDMA hydrogel was prepared by adding 90% (w/v) pyrolytic graphite powder into 20% (w/v) PEGDMA prepolymer solution, and vortexing for 1 min. The prepolymer solution was pipetted onto 1 × 1 cm 2 shape PMMA mold laid on a glass coverslip. Another coverslip was then placed upon the mold. The setup was exposed to UV light with optimized parameters: 5 cm between the setup and the light source, 6.9 W cm −2 UV intensity and 30 s crosslinking time. The gel was then placed into a PMMA chamber fabricated by laser cutter (VersaLaser, Scottsdale AZ) and assembled by epoxy (2 Ton, Cleaer Epoxy, In DevTube). PBS mixed with OptiPrep was prepared as a pre-solution of paramagnetic medium. 300 mg ml −1 stable radical was then added to the pre-solution, forming 1.8 M radical solution to provide a levitation environment for gels. Gel fabrication for Supplementary Movie 2 . Two pyrolytic graphite-embedded square PEGDMA gels were fabricated (the same size and component as those in Supplementary Movie 1 ). Two 1 × 1 cm 2 gels were incubated separately in 0.6 M (the gel at left) and 6 M radical solution (gel at right) for overnight. After magnetization, the gels were picked up and place within 0.16 M Gd solution in PMMA chamber for the levitation. The Gd solution was prepared by adding gadolinium salt into PBS, vortexing for 1 min, and then incubated in 80 °C oven for 20 min. Gel fabrication for Supplementary Movie 3 . Pyrolytic graphite-embedded PEGDMA hydrogel was prepared by adding 90% (w/v) pyrolytic graphite powder, into 20% (w/v) PEGDMA prepolymer solution and vortexed for 1 min. The mixed prepolymer solution was then pipetted onto a 600-μm spacer, then covered by a coverslip. A photomask (1 × 1 mm square shape) was placed onto the coverslip. The whole setup was exposed to the UV light with optimized parameters: 5 cm between the setup and the light source, 6.9 W cm −2 UV intensity, and 25 s crosslinking time. Individual square PEGDMA gel blocked was picked up. Ten of the gels were stained with blue colour and incubated in 6 M radical solution, whereas another ten gels were stained in yellow and incubated in 0.6 M radical solution. In both cases, the gels were incubated overnight. After magnetization, gels were placed within 0.191 M Gd solution in PMMA chamber for the levitation. The Gd solution was prepared by adding gadolinium salt into PBS, vortexing for 1 min and then incubated in 80 °C oven for 20 min. How to cite this article: Tasoglu, S. et al. Guided and magnetic self-assembly of tunable magnetoceptive gels. Nat. Commun. 5:4702 doi: 10.1038/ncomms5702 (2014).